Bio-inspired networks for optoelectronic applications Modern optoelectronics needs development of new materials characterized not only by high optical transparency and electrical conductivity, but also by mechanical strength, and flexibility. Recent advances employ grids of metallic micro- and nanowires, but the overall performance of the resulting material composites remains unsatisfactory. In this work, we propose a new strategy: application of natural scaffoldings perfected by evolution. In this context, we study two bio-inspired networks for two specific optoelectronic applications. The first network, intended for solar cells, light sources and similar devices, has a quasi-fractal structure and is derived directly from a chemically extracted leaf venation system. The second network is intended for touch screens and flexible displays, and is obtained by metalizing a spider’s silk web. We demonstrate that each of these networks attain an exceptional optoelectonic and mechanical performance for its intended purpose, providing a promising direction in the development of more efficient optoelectronic devices. The advent of optoelectronics in the 1950s has depended on the development of transparent conductors [1] . Such electrically conducting and optically transparent materials play a critical role in numerous important optoelectronic devices such as photovoltaic sensors, solar cells, photo diodes and lasers, all of which harvest or emit light. However, high optical transmission and good electrical conductivity are mutually limiting requirements since electrical carriers invariably scatter photons, and require a compromise. One successful approach had been to exploit the fundamental property of any carrier plasma, electromagnetic transparency above its plasma frequency. This idea led to the development of an entire class of materials (metal-oxides), which dominate the field today, such as the ubiquitous indium tin oxide (ITO), a metal with the plasma frequency in the infrared range, and thus transparent in the visible range [2] . However, while metal-oxides often have desirable electro-optical properties, they are also brittle, and this deficiency limits their usefulness in many practical applications. To address these challenges, new approaches have been recently devised, based on metallic micro- and nanoscaffoldings (such as wire and nanowire grids [3] , [4] , [5] , [6] , [7] , [8] , [9] , [10] , nanoparticles [11] , [12] and so on) and even using atomic-scale scaffolds such as graphene [13] , [14] . Structures of this kind do in fact improve mechanical flexibility, but their electro-optical performance has not yet been sufficiently high. In this work, we propose a new strategy, based on adopting ingenuous network designs readily found in nature. Indeed, micro- and nanoscaffolds of exceptional properties occur naturally in many biological systems, generated by a genetic code of a given organism, and self-assembled during the organism development [15] , [16] , [17] . These structures perform various functions, such as a support for mechanical cellular integrity (for example, nanoscopic cellular cytoskeletons) [18] , nutrients distribution via microfluidic channels (for example, leaf or insect wing venations) [19] , [20] , light management (for example, the Moth eye) [21] , improved mobility (for example, shark skin microtextures) [22] , [23] , [24] , super-hydrophobic behaviour (Lotus leaf) [23] , antibacterial protection (cicada wings) [25] and so on. Some of the most ingenious man-made material designs, such as velcro [23] , have effectively ‘copied’ existing solutions in nature. Moreover, most of these solutions have been undergoing a natural process of an evolutionary optimization for millions of years. In this work, inspired by such biostructures, we develop two distinct highly conducting and transparent microscaffold networks, each satisfying different requirements dictated by a specific application. We demonstrate that these networks show exceptional performance, outperforming most other recently proposed micro- and nanoscaffold schemes. The first network, to be employed as a window electrode for solar cells, light sources (for example, light-emitting diode), transparent heaters and so on, is obtained by metallization of a leaf venation (LV), a natural microfluidic network structure present in all leafs. This structure has been modified by evolution (at each generation) towards the optimized function of efficient delivery of nutrients to every cell of a leaf from a central vein, with very low light shading. The result of this natural optimization process is a quasi-fractal (or hierarchical) structure of LV [26] . Even though the process of this evolutionary optimization still continues, as evidenced by the variety of the existing LV structures today, the natural quasi-fractal structures are expected to be close to the optimum. Indeed, striking similarities have been observed for natural and optimal networks (obtained by computationally minimizing the total rate of energy expenditure), in their fractal aggregation structure [27] . This implies, that a whole class of natural hierarchical (quasi-fractal) structures exist, which are close to optimum, that is, each can be considered an approximately optimal network. Note that the question whether strictly fractal structures are indeed optimal, continues to be debated [28] , [29] , [30] . The key justification for employing the metalized near-optimal LV network as an efficient electrode, is the assumption that the electrical current flow properties of this structure are analogous to those of fluid. Indeed, the electric current flow is described by the Laplace equation, and so is the inviscid, incompressible and irrotational fluid flow [31] . Thus, even though not strictly optimal, the metallized, quasi-fractal LV networks are expected to outperform the uniform networks, as well as the primitive hierarchical bar-finger structures (often used) in solar cells, light sources and other similar applications. The second network, to be employed in various display applications (including touch screens and flexible displays), is obtained by metallizing a common silk spider web (SSW), a natural insect trap, made of nearly invisible, nanoscopically thin threads of exceptional mechanical strength and elasticity [32] . LV networks For the LV network, we have chosen the plant Magnolia alba (common name White Jade Orchid Tree). This abundant plant has leaves about 20 cm in length, of lanceolate shape and prominent secondary veins paired oppositely (pinnate venation), see Fig. 1a . From these secondary veins emanate smaller veins forming an angular network (reticulate veins). Insets in this figure show subsequent magnifications of the dotted area, with the finest, chemically extracted microstructure of the network shown in the scanning electron microscope (SEM) image ( Fig. 1b ). The smallest veins have diameter of about 50–110 μm, and are split into two shorter branches at each node. Networks of this kind, called ‘umbrella trees’, are non-uniform fractals, whose fractal properties pertain to the ‘canopy,’ that is, to the structure formed by the tips of the branches rather than the whole pattern [33] . The difficulty in characterizing the structure shown in Fig. 1b , and determining its approximate fractal dimension using the standard method based on branch ordering taxonomy [34] , [35] is the irregular nature of the venation network, which leads to large uncertainty in the measurements. An alternative approach, proposed here, is to consider angles between subveins at each bifurcation level, which are relatively easy to measure. Umbrella canopies usually display a particular branching angle for a given magnification ratio, namely the smallest angle compatible with self-avoidance (in two dimension), as discussed in ref. 33 . Since the fractal dimension is a nearly linear function of the branching angle ϑ B , based on data taken from plate 155 in ref. 33 , it is easy to convert ϑ B into the fractal dimension D S . Using five prominent nodes in Fig. 1a yields ϑ B =110±10 o , and, accordingly, D s =1.4±0.2. This value is consistent with the typical range 1.4–1.8 as reported in ref. 36 , and thus confirms that the network is an approximate non-uniform fractal. Note that the maximal distance between veins is much less than 1,000 μm, much smaller (better for current extraction) than in the conventional, commercial c-Si solar cells. The fabrication process for the LV metallic network skeleton is shown in Fig. 1c . It involves three steps: removing mesophyll while leaving the vein structure of the leaf intact by alkali solution etching [37] , metal coating (by silver sputtering) and transferring the network onto a chosen substrate, which could be glass, polymer or semiconductor. With a proper care, good adhesion could be assured. 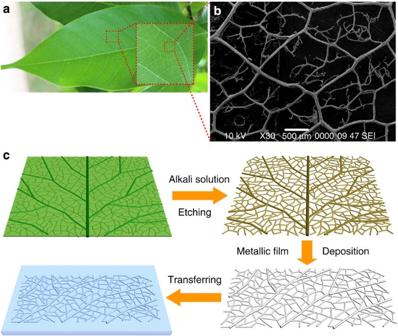Figure 1: Morphology and extraction of LV network. (a) Optical and (b) SEM images of the leaf and its LV network. (c) Schematic of the LV network fabrication method. The scale bar inbis 500 μm. Figure 1: Morphology and extraction of LV network. ( a ) Optical and ( b ) SEM images of the leaf and its LV network. ( c ) Schematic of the LV network fabrication method. The scale bar in b is 500 μm. Full size image Spider web networks For the SSW network, we have chosen a common spider Agelena labyrinthica , since its web has a distinct two-dimensional character, ideal for planar electrodes. 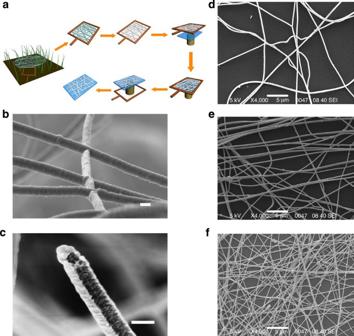Figure 2: Morphology and harvesting of the SSW. (a) Schematic of the fabrication process. (b) High-resolution SEM image of a small area of the network. (c) High-resolution SEM image of a single fibre of the network. (d–f) SEM images of one, two and four layers of the SSW network, respectively. The scale bars inbandcare 100 nm and ind–f, 5 μm. Figure 2a shows schematically the processes of the SSW-based silver network fabrication, which includes three steps: collecting SSW onto a sample holder, metal coating (Ag sputtering) and finally transferring the SSW network onto a substrate. Figure 2: Morphology and harvesting of the SSW. ( a ) Schematic of the fabrication process. ( b ) High-resolution SEM image of a small area of the network. ( c ) High-resolution SEM image of a single fibre of the network. ( d – f ) SEM images of one, two and four layers of the SSW network, respectively. The scale bars in b and c are 100 nm and in d – f , 5 μm. Full size image The micro- and nanomorphology of this network is demonstrated with SEM images in Fig. 2b–f . This is a nanostructure, with diameters of individual threads of the order of 100 nm, and the inter-thread spacing of the order of a few microns. Figure 2c shows an incomplete core-shell structure: silk core (~80 nm diameter), coated with an ~40-nm thin layer of silver. AFM image of the silver SSW network, and the corresponding AFM profile are shown in Supplementary Fig. 1 . Electro-optical performance The electro-optical properties of LV and SSW networks are summarized in Fig. 3a , which presents the transmittance ( T ) versus sheet resistance ( R s ) measurements, compared with those of other networks reported in the literature [4] , [5] , [6] , [7] , [8] , [9] , [10] , as well as the conventional transparent conducting electrode material ITO. Transmittance represents percentage of the light flux transmitted across the sample at a given frequency (or vacuum wavelength, here chosen to be λ =550 nm). The sheet resistance is the resistance (at zero frequency) of a square of a thin film of thickness d , measured from side-to-side, also given by R S = ρ / d , where ρ is the material resistivity. The data displayed are also quantified by using the so-called figure of merit, defined as [4] , [13] F = σ dc / σ opt , where σ dc =1/ ρ is the electrical conductance at zero frequency and σ opt is the electrical conductance measured in the optical frequency range (typically at the vacuum wavelength λ =550 nm). 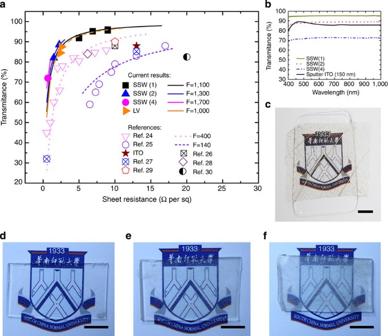Figure 3: Optoelectronic performance of LV and SSW networks. (a) Comparison with other networks and ITO (~150 nm) at the vacuum wavelength of 550 nm. The lines represent fits of equation (1) to the clusters of data points, which determine the corresponding figures of meritF. The error bars are smaller than the symbol sizes. (b) Transmittance versus radiation wavelength for the SSW networks and the standard, 150-nm thick ITO film. (c,d) Demonstration of the networks optical transparency for the LV, SSW(1), SSW(2) and SSW(4) networks, respectively. SSW(1), SSW(2) and SSW(4) denote the SSW network films with one, two and four layers, respectively. The scale bars inc–fare 1 cm. It has been shown [13] that F is simply related to T and R S via Figure 3: Optoelectronic performance of LV and SSW networks. ( a ) Comparison with other networks and ITO (~150 nm) at the vacuum wavelength of 550 nm. The lines represent fits of equation (1) to the clusters of data points, which determine the corresponding figures of merit F . The error bars are smaller than the symbol sizes. ( b ) Transmittance versus radiation wavelength for the SSW networks and the standard, 150-nm thick ITO film. ( c , d ) Demonstration of the networks optical transparency for the LV, SSW(1), SSW(2) and SSW(4) networks, respectively. SSW(1), SSW(2) and SSW(4) denote the SSW network films with one, two and four layers, respectively. The scale bars in c – f are 1 cm. Full size image Thus, F can be simply determined by fitting equation (1) to the data points for a given network, with F as the fitting parameter. These fits are shown in Fig. 3a as lines, and the corresponding extracted F ’s are indicated in the legend. Clearly, larger figure of merit F corresponds to more efficient networks. Our SSW networks are represented in Fig. 3a as solid squares (single layer), blue triangles (two layers) and solid circles (four layers) and our LV networks by orange right-pointing triangles (colour online). All our networks show superior performance, with the record high figures of merit, in the range F =1,000 to 1,700, and the four-layer SSW network reaching approximately F =1,700. Note that all the other reported uniform networks (based on nanowires, nanotroughs, nanocracks and so on) have much smaller figure of merit in the range F <400. In particular, our networks are superior to the industry standard ITO. This is further illustrated in Fig. 3b , which shows transmittances versus wavelength for our SSW-based networks and for the standard, 150-nm thick ITO film. Clearly, a single layer of our SSW network is ~10% more transparent, and by a factor of ~2 more conducting than the ITO film. Two layers of this network are equally transparent, but six times less resistive than ITO. Our LV network has also a very high figure of merit, F =1,000, even though its quasi-fractal structure is not far from optimal for current delivery but not necessarily for minimizing the total sheet resistance. To account for the LV network quasi-fractal structure, we have also measured resistances of the LV, as well as the uniform (non-hierarchical) SSW and the ‘crack’ [4] networks, adjusted to have all identical transmittances (of about 85%), and with the sample contacts configuration chosen so that the main vein of the LV network and its local, highly bifurcated region were contacted. The same contact configuration was also used for the SSW and ‘crack’ networks. The resulting resistance of the LV network has been found to be reduced by the factors of 0.81 and 0.61 compared with the SSW and the ‘crack’ networks, respectively, clearly demonstrating the advantage of the quasi-fractal structure for a directed current transport. Figure 3c–f shows optical images of the LV network, as well as one, two and four layers of the SSW network, respectively. Photographs were taken with the networks placed against a printed logo to visualize transparency. Even though the LV network is very transparent, the large-scale veins clearly visible in the inset of Fig. 3c make this network not suitable for display applications. However, in addition to solar cell and light source applications, LV network also can be used as a transparent film heater. Such a heater is demonstrated in the Supplementary Fig. 2 . Elastic properties We now address elastic properties of the networks. 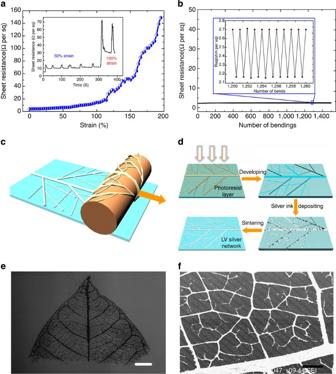Figure 4: Elastic properties of the SSW and replication of the LV networks. (a) SSW network sheet resistance (after tension release) versus strain. The error bars are smaller than the symbols. The inset shows time evolution of the network resistance subject to a train of eight stretching pulses: 50% strain (first six pulses), 100% strain (last two pulses). (b) SSW sheet network resistance versus repeated elastic bending events (180°, 1 mm radius). Inset: a zoomed-in fragment of the main curve showing perfectly repeatable sheet resistance oscillations, even after over one thousand bending events. (c) Schematic of the drum printing of the LV network. (d) Schematic of the photolithographic printing of the LV network. (e) Silver ink print of the LV network. (f) Contact photolithography of the LV network. The scale bars foreandfare 1 cm and 500 μm, respectively. Figure 4a is a plot of the SSW network resistance (after tension release) versus strain. Three ranges can be identified. In the elastic range (strains smaller ~25%), the original network resistance is repeatedly and fully recovered after each strain. In the reversible range (for larger strains, but smaller than ~100%), for multiple stretching the sample returns repeatedly the same value of the total resistance. For strains larger than ~100% (irreversible range), repeated stretching leads to the overall increase of the total resistance. The inset in Fig. 4a shows time evolution of the network resistance subject to a sequence of eight stretching pulses, each located at the beginning of the corresponding peak. The first six correspond to 50% and the last two to 100% strain pulses. The microscopic investigation of the samples clarifies this behaviour. In the elastic range, stretching of the SSW network breaks no fibres, since they are quite loose (see Fig. 2d ), with very few fibres fully stretched. The stretching therefore simply straightens the fibres, which causes only minimal damage of the metal coating. In the reversible range, stretching breaks some fraction of the fibres, which causes an increase of the total resistance. However, if the strain is limited to the same level at each subsequent stretching, no further breaking of fibres occurs, and resistance repeatedly returns to the same value. Finally, in the irreversible range, a large number of fibres, as well as the coating, become broken, while the remaining are near the breaking point, irreversibly affecting resistance of the metallic coating. The network conduction becomes unstable, very sensitive to stretching and fluctuates with every stretch. SSW network is therefore shown to have excellent stability only in the elastic range. Figure 4b further confirms this by demonstrating network’s resilience to repeated elastic bending; its resistance changes reversibly from 2.2 to 2.7 Ω (180°, 1 mm bending radius), even after 1,500 bending events. Due to these remarkable properties, SSW-based networks could be used in touch screen displays and stretch sensors. A touch-screen device based on a SSW network is demonstrated in the Supplementary Fig. 3 . Figure 4: Elastic properties of the SSW and replication of the LV networks. ( a ) SSW network sheet resistance (after tension release) versus strain. The error bars are smaller than the symbols. The inset shows time evolution of the network resistance subject to a train of eight stretching pulses: 50% strain (first six pulses), 100% strain (last two pulses). ( b ) SSW sheet network resistance versus repeated elastic bending events (180°, 1 mm radius). Inset: a zoomed-in fragment of the main curve showing perfectly repeatable sheet resistance oscillations, even after over one thousand bending events. ( c ) Schematic of the drum printing of the LV network. ( d ) Schematic of the photolithographic printing of the LV network. ( e ) Silver ink print of the LV network. ( f ) Contact photolithography of the LV network. The scale bars for e and f are 1 cm and 500 μm, respectively. Full size image Scale and scalability Even though both LV and SSW networks are clearly good candidates for applications, the scalability and associated with that costs must be assessed. The structure of the LV network could be simply and massively replicated by printing. A schematic of a possible method is shown in Fig. 4c , where an LV network pattern is engraved on a drum, allowing large-scale roll-to-roll printing of the pattern on flat substrates. Figure 4d provides a schematic of the LV network replication by using a contact photolithography; this method could be used to engrave the drum shown in Fig. 4c . Figure 4e is an image of an LV network printed directly from the LV in silver ink on paper. This was achieved by attaching LV directly to a metallic block, and then using it as a stamp. The resolution of the stamped image is very good, with most features reproduced. Because of the relatively large size of the features in the LV network, photolithography can be employed as a part of the engraving procedure. Figure 4f shows an image of the photolitographically obtained LV network print (details in Supplementary Fig. 4 ). While such LV networks would be relatively easy and inexpensive to replicate on a large scale, a method to do the same for the SSW networks must yet be invented. A possible practical way could be to base the SSW-like network on inexpensive polymers (for example, Kevlar nanofiber, nanocellulose and so on). In conclusion, we have developed two different metallic networks for specific applications, inspired by, and employing natural network structures. The first network, designed for solar cells, light sources and surface heaters, exploits the fractal properties of LV systems. This network achieves superior current delivery to, and extraction from, a substrate, with minimal optical shading. The second network, envisioned for display applications and based on a spider web, was demonstrated to have outstanding electro-optical and mechanical properties, strength and flexibility. In particular, these two nature-inspired structures outperform all electrode systems and optoelectronic networks devised here-to-fore. Leaf etching by alkali solution The 0.1 g ml −1 NaOH solution (lab prepared) was used for etching. Magnolia alba leaves were immersed in the solution at 50–70 °C for 3 h. By continually tapping the softened leaf, the mesophyll was removed leaving the vein structure of the leaf intact. This procedure was followed by washing and drying. Ag and ITO film depositions Sputtering (AJA International. ATC Orion 8, USA) was used to deposit Ag and ITO films. The SSW and LV structures were placed in vacuum chambers, and the sputtering was performed at ~50 °C to avoid damaging the samples. Performance measurements Morphologies of samples were characterized in a SEM system (JEOL JCM-5700, Tokyo, Japan), and by employing an optical microscope (MA 2002, Chongqing Optical & Electrical Instrument Co.). The sheet resistance of samples was measured by employing the standard van der Pauw method. Four contacts were deposited at the corners of a square sample (2 × 2 cm), numbered clockwise 1–4, and I–V data were recorded with the Keithley 2400 Source meter. Sheet resistance was calculated from the usual formula: R ab,cd =4.5( R 12,34 + R 34,12 + R 14,23 + R 23,14 )/4, with R ab,cd = U ab / I cd and where U ab is the voltage drop between ‘a’ and ‘b’ contacts, produced by current I cd flowing from contact ‘c’ to contact ‘d’. The second method, employed when the van der Pauw could not be used (for example, while the sample was stretched) was the two-probe method. In this method, two parallel electrodes (sputtered narrow silver lines of length L ) were placed on the surface of the sample. Sheet resistance was calculated from R s = R * L / W , where R is the measured resistance and the sample width is W . A modified two-probe method was also used for the directed current transport in the LV network, in which one electrode was a narrow line, and the other was a circular silver contact. In this case, a simple resistance between the electrodes was measured. To test the flexibility of SSW and LV networks, the structures were transferred to elastic substrates, for example, PDMS (Polydimethylsiloxane) and PET (polyethylene terephthalate). A lab-made stretching and bending system was used, with an automatic control and a data acquisition system. Optical transmittance was measured in an integrating sphere system (Ocean Optics, USA). These measurements were normalized to the absolute transmittance of the substrate (glass, PET or PDMS). How to cite this article : Han, B. et al . Bio-inspired networks for optoelectronic applications. Nat. Commun. 5:5674 doi: 10.1038/ncomms6674 (2014).